A novel pathway producing dimethylsulphide in bacteria is widespread in soil environments The volatile compound dimethylsulphide (DMS) is important in climate regulation, the sulphur cycle and signalling to higher organisms. Microbial catabolism of the marine osmolyte dimethylsulphoniopropionate (DMSP) is thought to be the major biological process generating DMS. Here we report the discovery and characterization of the first gene for DMSP-independent DMS production in any bacterium. This gene, mddA , encodes a methyltransferase that methylates methanethiol and generates DMS. MddA functions in many taxonomically diverse bacteria including sediment-dwelling pseudomonads, nitrogen-fixing bradyrhizobia and cyanobacteria, and mycobacteria including the pathogen Mycobacterium tuberculosis. The mddA gene is present in metagenomes from varied environments, being particularly abundant in soil environments, where it is predicted to occur in up to 76% of bacteria. This novel pathway may significantly contribute to global DMS emissions, especially in terrestrial environments and could represent a shift from the notion that DMSP is the only significant precursor of DMS. Globally, microbes, and particularly bacteria in the oceans and their margins, drive the production of dimethylsulphide (DMS), generating ~3 × 10 14 g of this gas per annum [1] through biotransformations of organosulphur molecules [2] , [3] . Much of the DMS produced is either catabolized by bacteria or photochemically oxidized [4] . However, ~10% escapes into the atmosphere making it the most abundant biogenically derived form of sulphur transferred from the sea to the air [4] . DMS oxidation products can act as cloud condensation nuclei, aiding cloud formation and affecting atmospheric chemistry [2] , [5] . This in turn can influence climate regulation [5] , although its significance has recently been questioned [6] . DMS is also a signalling molecule used by some seabirds, crustaceans and marine mammals as a foraging cue [7] . Marine DMS is produced predominantly as a result of microbial catabolism of the algal osmolyte dimethylsulphoniopropionate (DMSP) through the action of DMSP lyase enzymes [3] , [8] . However, there are microbial DMSP-independent pathways generating DMS that are not limited to marine environments, such as the enzymatic degradation of S-methyl-methionine, dimethyl sulphoxide (DMSO) or methoxyaromatic compounds [9] . Also, many varied anoxic environments produce DMS at levels (for example, 1–44 nM) [10] that can be in excess of those described for the upper marine water column [11] , possibly through microbial methylation of methanethiol (MeSH) [9] , [12] , a product of hydrogen sulphide (H 2 S) methylation, or methionine (Met) catabolism. These environments include freshwater lake sediments [10] , [13] , saltmarsh sediments [14] , cyanobacterial mats [15] and peat bogs, the latter of which cover 4 million km 2 worldwide and can emit ~6 μmol DMS m −2 per day [12] . The ability to generate MeSH from sulphide and/or Met under oxic conditions is common in heterotrophic bacteria from many diverse environments [16] , but to our knowledge there are no reports of aerobic bacteria generating DMS by MeSH methylation reactions in any environment. Thus, before this study, the significant levels of DMS produced by non-marine environments were apportioned solely to anaerobic microbes. Here we identify bacteria producing DMS, independent of DMSP, under aerobic conditions, and characterize the first gene for the production of DMS from MeSH in these bacteria. 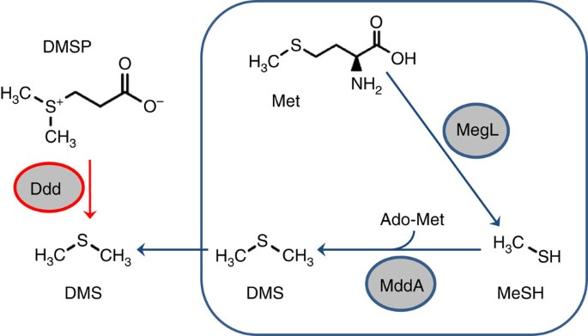Figure 1: A schematic representation of DMSP-dependent and MeSH-dependent DMS production pathways. Blue arrows signify pathways occurring inPseudomonas deceptionensisM1T, shown as a blue box. The red arrow signifies the DMSP cleavage pathway, present in some bacteria, that is catabolised by DMSP lyase enzymes (Ddd) and generates DMS. The amino acid Methionine (Met) is converted to MeSH by the Met gamma lyase enzyme (MegL) inP. deceptionensisM1T. The MddA enzyme methylates MeSH to DMS using Ado-Met as the methyl donor. DMS production by Pseudomonas deceptionensis M1 T We noted that Pseudomonas deceptionensis M1 T , a new species isolated from Antarctic marine sediment [17] , produced DMS from minimal media containing magnesium sulphate as the only sulphur source ( Table 1 ). P. deceptionensis M1 T does not synthesize DMSP, nor does it catabolize DMSP with its genome lacking any known genes for DMSP catabolism [3] , [8] . Therefore, P. deceptionensis M1 T has a novel DMSP-independent DMS production pathway. Table 1 The DMS and MeSH produced by key microbial strains used in this study. Full size table In P. deceptionensis M1 T , Met and MeSH are precursors for DMS since both these molecules significantly enhanced (four- to sevenfold) DMS production, with MeSH also being produced from Met ( Table 1 ). The P. deceptionensis M1 T genome contains a homologue of the megL gene, whose Met gamma lyase product (EC4.4.1.11) would be predicted to cleave Met to MeSH. A P. deceptionensis M1 T megL mutant strain (J565) was constructed and found to no longer make MeSH or DMS from either minimal medium or medium supplemented with Met ( Table 1 ). However, the megL mutant strain did make DMS when exogenous MeSH was added, supporting the pathway proposed in Fig. 1 , namely that the direct precursor for DMS was MeSH, this reaction being mediated via an enzyme activity that we termed Mdd, for MeSH-dependent DMS. Figure 1: A schematic representation of DMSP-dependent and MeSH-dependent DMS production pathways. Blue arrows signify pathways occurring in Pseudomonas deceptionensis M1 T , shown as a blue box. The red arrow signifies the DMSP cleavage pathway, present in some bacteria, that is catabolised by DMSP lyase enzymes (Ddd) and generates DMS. The amino acid Methionine (Met) is converted to MeSH by the Met gamma lyase enzyme (MegL) in P. deceptionensis M1 T . The MddA enzyme methylates MeSH to DMS using Ado-Met as the methyl donor. Full size image Identification of the mddA gene To identify the mdd gene(s) responsible for the conversion of MeSH to DMS, a genomic library of P. deceptionensis M1 T was constructed in the wide host-range cosmid pLAFR3. This library was screened in the heterologous host Rhizobium leguminosarum and a clone, pBIO2219, was isolated that conferred the ability to produce DMS from MeSH at levels similar to that of P. deceptionensis M1 T itself ( Table 1 ). Using transposon mutagenesis, a Tn 5lac insertion in pBIO2219 was identified that abolished the Mdd + phenotype, and was mapped to a gene termed mddA . When cloned alone and expressed under the control of the T7 promoter in Escherichia coli , mddA conferred MeSH-dependent DMS production ( Table 1 ). Furthermore, an insertional mutation in mddA of P. deceptionensis M1 T (strain J566) completely abolished DMS production, without affecting the ability to produce MeSH from Met ( Table 1 ). DMS and MeSH production from H 2 S Given that it has been shown previously that MeSH is produced from H 2 S [16] , both P. deceptionensis M1 T and E. coli expressing mddA were tested for MeSH and DMS production in the presence of H 2 S, but neither produced increased levels of these gases when compared to controls without the addition of H 2 S. This suggests that H 2 S is not a significant contributor to DMS production through the MddA pathway in P. deceptionensis M1 T . MddA is a membrane methyltransferase The polypeptide sequence of MddA has no significant sequence identity to any characterized enzyme, but has limited similarity to S-isoprenylcysteine methyltransferases (COG2020, Fig. 2 ), supporting the proposed pathway ( Fig. 1 ), whereby MddA would be a methyltransferase converting MeSH to DMS. Isoprenylcysteine methyltransferases, for example, Ste14p of Saccharomyces cerevisiae , which is localized in endoplasmic reticulum membranes, catalyse the S -adenosyl- L -Met (Ado-Met)-dependent carboxyl methylation of proteins [18] . MddA is also predicted to be a membrane protein containing four to six membrane-spanning helices ( Supplementary Table 1 ). As with Ste14p, in vitro Mdd activity in cell extracts of both P. deceptionensis M1 T and E. coli expressing MddA (16,200±2,130 and 1,750±291 pmol DMS min −1 per mg protein, respectively) required Ado-Met as methyl donor for MeSH to be converted to DMS. Also, subcellular fractionation of P. deceptionensis M1 T showed that Mdd activity was only seen in the membrane fraction (6,170±1,370 pmol DMS min −1 ·per mg protein). 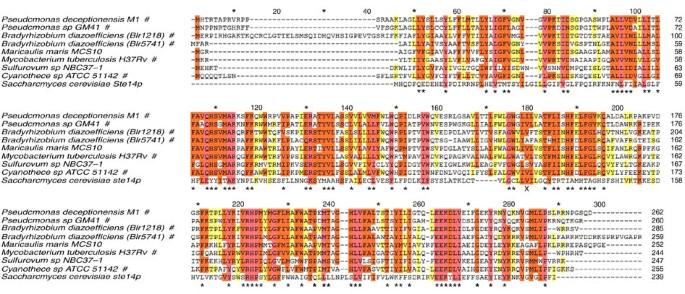Figure 2: ClustalW alignment of representative bacterial MddA polypeptides and theSaccharomyces cerevisiaeSte14p polypeptide. Residues that are identical or have similar properties are highlighted in red, orange or yellow if they are conserved in all nine, at least seven or at least five polypeptides, respectively. Residues with similar properties that are conserved in all eight bacterial MddA sequences are marked with asterisks below. The position of the Tn5lacZinsertion in thePseudomonas deceptionensis M1TmddAmutant J566 is marked with an ‘X’ below. Species names with the MddA polypeptide accession codes shown in brackets are:Cyanothecesp. ATCC 51142 (YP_001803274),Mycobacterium tuberculosisH37Rv (NP_217755),Bradyrhizobium diazoefficiensUSDA 110 (Blr1218; NP_767858.1),Bradyrhizobium diazoefficiensUSDA 110 (Blr5741, NP_772381.1),Pseudomonassp. GM41 (WP_008148420),Pseudomonas deceptionensisM1T(AJE75769),Maricaulis marisMCS10 (YP_757811.1),Sulfurovumsp. NBC 37-1 (YP_001358232.1). Species names marked with a hash indicate those MddA sequences whose activity has been ratified inEscherichia coli. TheSaccharomyces cerevisiaeSte14p accession is AAA16840.1. Figure 2: ClustalW alignment of representative bacterial MddA polypeptides and the Saccharomyces cerevisiae Ste14p polypeptide. Residues that are identical or have similar properties are highlighted in red, orange or yellow if they are conserved in all nine, at least seven or at least five polypeptides, respectively. Residues with similar properties that are conserved in all eight bacterial MddA sequences are marked with asterisks below. The position of the Tn 5lacZ insertion in the Pseudomonas deceptionensi s M1 T mddA mutant J566 is marked with an ‘X’ below. Species names with the MddA polypeptide accession codes shown in brackets are: Cyanothece sp. ATCC 51142 (YP_001803274), Mycobacterium tuberculosis H37Rv (NP_217755), Bradyrhizobium diazoefficiens USDA 110 (Blr1218; NP_767858.1), Bradyrhizobium diazoefficiens USDA 110 (Blr5741, NP_772381.1), Pseudomonas sp. GM41 (WP_008148420), Pseudomonas deceptionensis M1 T (AJE75769), Maricaulis maris MCS10 (YP_757811.1), Sulfurovum sp. NBC 37-1 (YP_001358232.1). Species names marked with a hash indicate those MddA sequences whose activity has been ratified in Escherichia coli . The Saccharomyces cerevisiae Ste14p accession is AAA16840.1. Full size image MddA functions in taxonomically diverse bacteria The MddA polypeptide is highly conserved in specific Pseudomonas species ( Figs 2 and 3 , and Supplementary Table 2 ). In every case tested, the presence of mddA in pseudomonads correlated with the strain producing DMS. Both Pseudomonas fragi DSM 3456 and Pseudomonas sp. 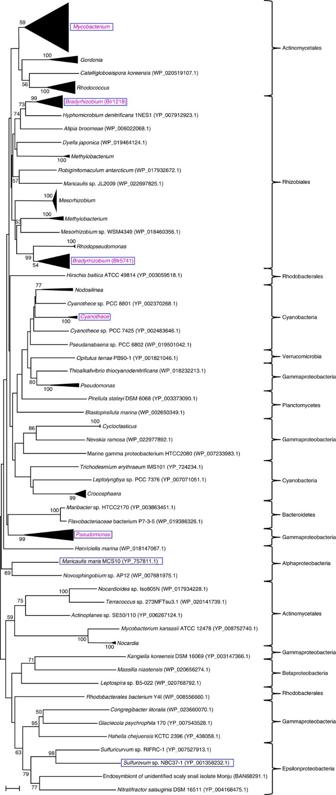Figure 3: Molecular phylogenetic analysis of MddA proteins. Bacterial strains, their taxonomy and the accession codes of bacterial MddA proteins that have >40% amino acid identity toPseudomonas deceptionensisM1TMddA are shown. Sequences with >57% identity to each other that are in bacteria of the same genus are shown with triangles; the size of the triangle reflects the number of sequences. Those cases where the clonedmddAgenes were shown experimentally to confer MeSH-dependent DMS production toEscherichia coliare written in purple. The two MddA proteins ofBradyrhizobium diazoefficiensUSDA 110 (Blr1218 and Blr5741) are shown. MddA sequences that were aligned inFig. 2are in blue boxes. The neighbour-joining tree shown was obtained using the Jones–Taylor–Thornton (JTT) model of amino acid substitution. Bootstrap values ≥50% (based on 1,000 replicates) are shown at branch points. The tree is drawn to scale, with branch lengths measured in the number of substitutions per site. The scale bar indicates 0.1 substitutions per site. GM41 showed DMS production rates similar to P. deceptionensis M1 T , which were also enhanced by MeSH ( Supplementary Table 3 ), and cloned mddA from Pseudomonas sp. GM41 conferred Mdd activity to E. coli ( Supplementary Table 3 ). The mddA gene in pseudomonads is located between genes that have either not been characterized in any organism or which have no known connection to sulphur metabolism ( Supplementary Fig. 1 ). Of the pseudomonads lacking mddA , for example, Pseudomonas putida and Pseudomonas psychrophila those tested showed no detectable levels of DMS production ( Supplementary Table 3 ). Figure 3: Molecular phylogenetic analysis of MddA proteins. Bacterial strains, their taxonomy and the accession codes of bacterial MddA proteins that have >40% amino acid identity to Pseudomonas deceptionensis M1 T MddA are shown. Sequences with >57% identity to each other that are in bacteria of the same genus are shown with triangles; the size of the triangle reflects the number of sequences. Those cases where the cloned mddA genes were shown experimentally to confer MeSH-dependent DMS production to Escherichia coli are written in purple. The two MddA proteins of Bradyrhizobium diazoefficiens USDA 110 (Blr1218 and Blr5741) are shown. MddA sequences that were aligned in Fig. 2 are in blue boxes. The neighbour-joining tree shown was obtained using the Jones–Taylor–Thornton (JTT) model of amino acid substitution. Bootstrap values ≥50% (based on 1,000 replicates) are shown at branch points. The tree is drawn to scale, with branch lengths measured in the number of substitutions per site. The scale bar indicates 0.1 substitutions per site. Full size image Importantly, MddA-like proteins are also present in a wide range of other bacterial taxa, including widely studied and important groups, and many which had not previously been suspected to make DMS. Proteins sharing ~50% amino acid sequence identity to P. deceptionensis M1 T MddA are present in multiple species of the actinobacteria Gordonia , Rhodococcus and Mycobacterium , including the pathogens M. tuberculosis and M. avium , Rhizobiales members including N 2 -fixing Mesorhizobium and Bradyrhizobium (two distinct forms, ~50% identical to each other, exist in many, for example, B. diazoefficiens USDA 110 Blr1218 and Blr5741) and N 2 -fixing cyanobacteria, including Cyanothece , Pseudanabaena and Nodosilinea species ( Figs 2 and 3 , and Supplementary Table 2 ). MddA-like proteins also exist, although less frequently, in some Planctomycetes, Flavobacteria, Spirochaetes, Verrucomicrobia and Alpha-, Beta-, Gamma- and Epsilonproteobacteria ( Figs 2 and 3 , and Supplementary Table 2 ). It is known that some mycobacteria that contain mddA produce DMS, including M. bovis BCG [19] , but no soil-dwelling Bradyrhizobium or cyanobacteria, have previously been reported to produce DMS. We found that B. diazoefficiens USDA 110 and Cyanothece sp. ATCC 51142 produced DMS when grown in minimal media and that this DMS production was enhanced by addition of MeSH ( Table 1 ). Our finding that some cyanobacteria are Mdd + may explain why DMS production observed in a freshwater lake coincided with cyanobacterial blooms [13] . The genes encoding the MddA polypeptides from B. diazoefficiens USDA 110 (blr1218 and blr5741, Rhizobiales), M. tuberculosis H37Rv (Actinomycetales) and Cyanothece sp. ATCC 51142 (Cyanobacteria), which form distinct clades of the MddA phylogenetic tree ( Fig. 3 ), were cloned and expressed in E. coli. In all cases, these genes gave significant Mdd activity, including both copies present in B. diazoefficiens USDA 110 ( Supplementary Table 3 ), perhaps explaining why this widely studied strain produces ~50-fold more DMS than other tested bacteria. We conclude that the mddA gene is widespread in taxonomically diverse bacteria, and that its occurrence in a bacterium is indicative of the capacity to generate DMS from MeSH. 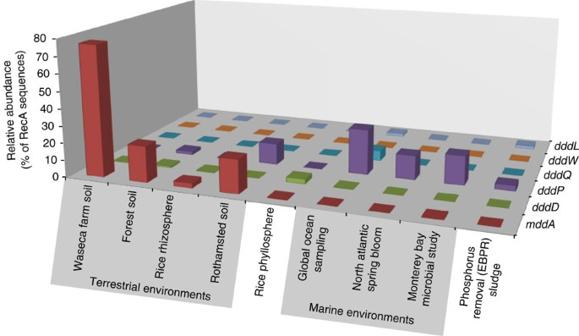Figure 4: Comparison of normalized values ofmddAanddddDPQWLsequences in different environmental metagenomes. Details of metagenomes are inSupplementary Table 4and the number of unique hits (Supplementary Table 5) were normalized to the number of unique RecA sequences in the metagenome and are presented as percentage of the total RecA sequences. Peptide databases were downloaded from metagenome sequences available from CAMERA and MG-RAST. RecA and Ddd probe sequences are detailed inSupplementary Table 6. mddA is particularly abundant in soil environments The environmental abundance of the mddA gene was estimated by probing metagenomic data sets from a range of environments ( Supplementary Table 4 ). MddA protein-encoding genes (E<e −30 ) were represented in most metagenomes, but strikingly were much more abundant in terrestrial environments, especially soil metagenomes, where mddA was predicted to be present in 5–76% of bacteria ( Fig. 4 , Supplementary Table 5 ). Interestingly, mddA was much less abundant in marine metagenomes where it only occurred in ≤0.5% of bacteria, in contrast to some ddd DMSP lyase genes, whose products produce DMS from DMSP and are much more abundant in marine metagenomes [8] ( Fig. 4 , Supplementary Table 5 ). Therefore, unlike previously identified DMS-producing enzymes, MddA is likely more important in the production of DMS from terrestrial rather than marine environments. Figure 4: Comparison of normalized values of mddA and dddDPQWL sequences in different environmental metagenomes. Details of metagenomes are in Supplementary Table 4 and the number of unique hits ( Supplementary Table 5 ) were normalized to the number of unique RecA sequences in the metagenome and are presented as percentage of the total RecA sequences. Peptide databases were downloaded from metagenome sequences available from CAMERA and MG-RAST. RecA and Ddd probe sequences are detailed in Supplementary Table 6 . Full size image Potential roles of the MddA pathway P. deceptionensis M1 T cannot use DMS, or its precursors Met and MeSH, as a carbon source. It also cannot use DMS as a sulphur source, but can use Met and MeSH. Therefore, to study why bacteria containing mddA might make DMS, the transcription of the mddA gene was examined using mddA - lac transcriptional fusions in P. deceptionensis M1 T and available microarray data from B. diazoefficiens USDA 110 and M. tuberculosis H37Rv. In P. deceptionensis M1 T mddA was constitutively expressed (giving ~70 Miller units of β-galactosidase activity) irrespective of the potential inducer molecule or environmental conditions tested (see Methods). From experiments reported for B. diazoefficiens USDA 110 and M. tuberculosis H37Rv, there were no conditions that significantly affected mddA gene expression, with the exception that in M. tuberculosis H37Rv the transcription of mddA was 4-fold induced by addition of the anti-tuberculosis drug thioridazine, which contains a methylated sulphur group [20] . In Sulfitobacter sp. EE-36, the DMSP lyase gene dddL is also constitutively expressed and it is proposed that DMS is generated as a signalling molecule [3] . This is a possible explanation for the existence of the Mdd pathway in P. deceptionensis M1 T and other Mdd + bacteria, since it is well documented that DMS is a chemoattractant [7] and in some environments may play a major role in structuring bacterial communities [21] . Many heterotrophic bacteria, including P. putida DS1 (ref. 22 ), oxidize DMS to DMSO, with some coupling this reaction to adenosine triphosphate synthesis and increased biomass production [23] , [24] . P. deceptionensis M1 T also generated DMSO, likely via the oxidation of DMS because estimates of DMSO production by the wild type strain (0.64 pmol DMSO min −1 per mg protein) were sevenfold higher than the mddA mutant. Oxidation of DMS to DMSO may form part of an antioxidant cascade protecting against oxidative stress [25] . However, in P. deceptionensis M1 T , it is unlikely that the MddA pathway has a role in protection against oxidative stress or energy production since the mddA mutant showed no growth deficiency when compared with the wild type under all tested conditions, including oxidative stress, and the expression of the mddA gene was also unaffected by oxidative stress. Another function for MeSH-dependent DMS production in these bacteria could be in regulating the levels of Met in the cell. If Met levels in the cell were to become too high, conversion to MeSH, and then subsequently DMS through the action of MddA, would provide a pathway for the removal of excess Met without leading to an accumulation of the potentially harmful MeSH [26] . However, while still possible, this idea is not supported by the fact that mddA transcription was unaffected by Met (see above) or that the mddA mutant showed no decreased tolerance to MeSH, at least under our conditions. The mddA gene encodes a methyltransferase that catalyses the conversion of MeSH into DMS and represents the first gene characterized for DMSP-independent DMS production in any bacterium. Although the role of the Mdd pathway in bacteria remains unclear, it is possible, given the distribution of mddA in taxonomically diverse bacteria and in varied environments, that this pathway may play a significant role in the global biogenic sulphur cycle. Also the relative abundance of mddA in terrestrial metagenomes, rather than marine metagenomes, indicates that DMS produced from non-marine, and critically non-DMSP, sources may play a more significant role in global DMS production than previously thought. Bacterial strains and culturing Strains and plasmids used in this study are shown in Supplementary Tables 7 and 8 . Pseudomonas deceptionensis M1 T , Pseudomonas sp. GM41, Pseudomonas fragi DSM 3456, Pseudomonas psychrophila DSM 17535, Pseudomonas putida ATCC 12623 and Escherichia coli strains were grown in LB (complete) and M9 (minimal) media [27] for 48 h at 28 °C and overnight at 37 °C, respectively. Bradyrhizobium diazoefficiens USDA 110 and Rhizobium leguminosarum J391 were grown in TY (complete) and Y (minimal) media [28] for 48 h at 28 °C. Cyanothece sp. ATCC 51142 was grown in ATCC 1047 media [29] , [30] at 26 °C under constant light conditions (50 μE m −2 s −1 ) for 1 week. Sole carbon source growth tests A culture of P. deceptionensis M1 T in M9 was washed three times with M9 without any carbon source and inoculated into fresh M9 media containing no carbon source, 10 mM glycerol or 5 mM DMSP (made in house [31] ), 5 mM Met (Sigma Aldrich), 2 mM DMSO (Sigma Aldrich), 1 mM DMS (Sigma Aldrich) or 1 mM MeSH (Sigma Aldrich) as the sole carbon source. Cultures were incubated at 28 °C for 5 days and growth was estimated by measuring the OD 600 of the cultures with a spectrophotometer UV-1800 (Shimadzu). Sole sulphur source growth tests Cultures of P. deceptionensis M1 T in M9 were washed three times with M9 without sulphur and inoculated into fresh M9 media containing no sulphur or MgSO 4 , DMSP, Met, DMSO, DMS or MeSH as the sole sulphur source at 100 μM concentrations. Cultures were incubated at 28 °C for 5 days and the growth was estimated by measuring the OD 600 of the cultures with a spectrophotometer UV-1800 (Shimadzu). General in vivo and in vitro genetic manipulations Plasmids were transferred either by conjugation from E. coli to R. leguminosarum J391 or P. deceptionensis M1 T J564 using helper plasmid pRK2013 (ref. 32 ); or by electroporation into P. deceptionensis M1 T J564 using a BIORAD MicroPulser machine as in Tombolini et al. [33] Bacterial genomic DNA was isolated using a Promega genomic preparation kit. Routine restriction digestions, ligations, Southern blotting and hybridizations were performed essentially as in Downie et al. [34] The oligonucleotide primers used for molecular cloning were synthesized by Eurofins Genomics and are detailed in Supplementary Table 9 . Sequencing of plasmids and PCR products was done by the dideoxy chain termination method by Eurofins Genomics. Sequencing of P. deceptionensis M1 T genomic DNA Generation of a draft genome sequence of P. deceptionensis M1 T is in progress. High molecular weight P. deceptionensis M1 T genomic DNA was extracted using a Qiagen genomic tip 100/G and Qiagen buffer set (Qiagen, Hilden, Germany). The genomic DNA was fragmented using Ion Shear reagents, followed by ligation with Ion Adapters, as described in the Ion Xpress Plus gDNA Fragmentation Library Preparation manual (Life Technologies Inc.). A 400-bp library was prepared by size selection of 450–500-bp fragments from a 2% agarose gel. The Ion sphere particles were templated using the Ion OneTouch 2 instrument with the Ion PGM Template OT2 400 Kit, and then enriched using the Ion OneTouch ES. Sequencing was performed on an Ion PGM Sequencer with an Ion 316 chip v2 and the Ion PGM Sequencing 400 Kit. The generated fastq file containing the resulting sequences was trimmed using Galaxy ( https://usegalaxy.org/ ). Ends were trimmed to remove all bases with quality scores less than 50 and all ambiguous bases from each end were trimmed. The remaining sequences were assembled using Lasergene (DNASTAR Inc.) and the default de novo assembly settings. The resulting contig sequences were analysed with Rapid Annotation using Subsystems Technology (RAST) [35] , Artemis v14.0.0 ( http://www.sanger.ac.uk/Software/Artemis ) and BioEdit [36] v7.1.3, and were searched for genes of interest by BLAST ( http://blast.ncbi.nlm.nih.gov/Blast.cgi ). The sequences of the cosmid clone insert from pBIO2219 and the megL gene have been submitted to the GenBank database (accession numbers KM030271 and KM030270, respectively). Mutation of the megL gene in P. deceptionensis M1 T For the targeted mutagenesis of the megL gene in P. deceptionensis M1 T , a 0.5-kb internal PCR fragment of megL ( Supplementary Table 9 ) was cloned into the suicide plasmid pBIO1879 (ref. 37 ) and transformed into P. deceptionensis M1 T J564 selecting for recombination on LB medium containing spectinomycin (800 μg ml −1 ) and kanamycin (20 μg ml −1 ). Genomic insertion mutations in P. deceptionensis M1 T J565 were confirmed by PCR. Construction of a P. deceptionensis M1 T genomic library P. deceptionensis M1 T genomic DNA was used to generate a genomic library in the cosmid pLAFR3 (ref. 38 ) as detailed in Curson et al. [39] Approximately 12,000 primary clones were obtained in E. coli 803 (ref. 40 ). A sample of 10 clones were characterized by restriction digestion and found to contain 25–35 kb inserts that all differed from each other. Screening of the P. deceptionensis M1 T genomic library The P. deceptionensis M1 T genomic library was mobilized en masse by triparental conjugation into R. leguminosarum J391 (ref. 41 ). Approximately 250 transconjugants, which arose on TY medium containing tetracycline (5 μg ml −1 ) and streptomycin (400 μg ml −1 ), were inoculated into 300 μl Y medium supplemented with 0.5 mM MeSH in 2 ml gas-tight vials (Alltech Associates) and were screened for DMS production, see below. Mutation of the mddA gene in P. deceptionensis M1 T The cosmid pBIO2219, which contains mddA and its surrounding region of P. deceptionensis M1 T genomic DNA, was mutagenized with Tn 5lacZ . pBIO2219 was transformed into E. coli strain A118 (ref. 42 ), then this transformant strain was used as the donor in a conjugational cross with R. leguminosarum J391. Derivatives of pBIO2219 with a Tn 5lacZ insertion in the cosmid were obtained by plating the cross on medium containing kanamycin (200 μg ml −1 ), streptomycin (400 μg ml −1 ) and tetracycline (5 μg ml −1 ). Individual colonies were inoculated into 300 μl Y medium supplemented with 0.5 mM MeSH, as above, and were screened for those derivatives that no longer produced DMS. The Tn 5lacZ insertion in pBIO2220 was precisely located within the mddA gene by sequencing. The pBIO2220 cosmid was transformed into P. deceptionensis M1 T J564 and then the mddA ::Tn 5lacZ mutation was introduced into the P. deceptionensis M1 T J564 genome by marker exchange, by conjugating in pPH1JI [43] (gentamycin resistant), the P1 group plasmid, to eliminate the pLAFR3-based cosmid, as in Downie et al. [34] Mutants were selected by their resistance to gentamicin (5 μg ml −1 ), kanamycin (20 μg ml −1 ) and sensitivity to tetracycline and were confirmed by PCR and Southern hybridization. Analysis of volatile organic sulphur compounds and DMSO P. deceptionensis M1 T wild type and J566 were grown on tryptone soya agar (Oxoid) slants in 20 ml gas chromatography headspace vials (Chromlab) for 72 h at 15 °C. Volatile organic sulphur compounds and DMSO produced were identified by solid-phase microextraction using a carboxen-polydimethylsiloxane fibre (CAR/PDMS, Supelco) coupled to gas chromatography—mass spectrometry (Trace GC Ultra+DSQII, Thermo Scientific) and a capillary column 1.8 μm DB-624 (60 m × 0.32 mm, Agilent Technologies). DMSP production and consumption assays P. deceptionensis M1 T was grown in M9 media in the presence and absence of 1 mM DMSP at 28 °C for 24 h. The culture was then pelleted and the supernatant was analysed for DMSP versus buffer control samples via the addition of 10 M NaOH to dilutions in gas-tight 2 ml vials (12 × 32 mm, Alltech Associates) and the subsequent liberation of DMS was quantified by gas chromatography, as below. Assays of microbial DMS and MeSH production To measure DMS and MeSH production in pseudomonads, R. leguminosarum , B. diazoefficiens and Cyanothece sp. ATCC 51142, each strain was first grown overnight (1 week for Cyanothece sp. ATCC 51142) in its appropriate minimal medium and, where indicated, 5 mM DMSP, 0.5 mM MeSH, 5 mM Met or 1 mM H 2 S. For Cyanothece sp. ATCC 51142, 300 μl of cultures were harvested and resuspended in the same volume of fresh media in sealed 2 ml vials and incubated overnight at 26 °C, as above, before being assayed for DMS and MeSH production. All other bacterial cultures were adjusted to an OD 600 of 0.3 and the cells were diluted 10-fold into 300 μl of minimal media supplemented with the additives as indicated above and incubated overnight at 28 °C in 2 ml vials before assaying for DMS. DMS and MeSH production in the headspace of vials was quantified by gas chromatography, using a flame photometric detector (Agilent 7890A GC fitted with a 7693 autosampler) and a HP-INNOWax 30 m × 0.320 mm column (Agilent Technologies J&W Scientific) capillary column. The detection limits for DMS and MeSH were 0.15 and 4 nmol, respectively. An eight-point calibration curve of DMS and MeSH standards was used as in Curson et al. [44] The protein content in the cells were estimated by a Bradford method (BioRad) and rates of MeSH and DMS production were expressed as pmol min −1 mg protein. MddA activity assays in P. deceptionensis M1 T cell lysates P. deceptionensis M1 T was grown in LB media for 24 h at 28 °C and 2 ml cell aliquots were pelleted, and resuspended in 500 μl of cold Tris 100 mM, MES 50 mM, acetic acid 50 mM (pH 7) buffer. Cell suspensions were sonicated (5 × 10 s) using an ultrasonic processor VC50 sonicator (Jencons) and the cell debris was pelleted. Triplicate 50 μl aliquots of the cell lysates were incubated with 1 mM Ado-Met and 1 mM MeSH for 2 h before quantifying the DMS produced in the headspace and protein concentrations, as above. Cell fractionation and MddA activity assays P. deceptionensis M1 T was grown in LB media for 24 h at 28 °C. After that period, 2 ml aliquots were fractionated into the periplasmic, cytoplasmic and membrane fractions using a PeriPreps Periplasting Kit (Epicentre) as in Curson et al. [45] Triplicate 50 μl of each fraction were incubated with 1 mM Ado-Met and 1 mM MeSH for 2 h before quantifying the DMS produced in the headspace of the vials and protein concentrations, as above. Assays of MddA activity in E. coli E. coli BL21 strains containing cloned mddA genes were grown at 37 °C in 5 ml of LB broth containing ampicillin (100 μg ml −1 ) to an OD 600 of 0.8. The cells were diluted 10-fold into 300 μl of M9 media containing 100 μM isopropyl β- D -1-thiogalactopyranoside and 0.5 mM MeSH or 1 mM H 2 S in 2 ml vials. Vials were incubated at 28 °C for 18 h and then DMS, MeSH and protein concentrations were assayed as above. E. coli cell lysate activity assays For cell lysate experiments, E. coli BL21 containing cloned mddA genes were grown to an OD 600 of 0.4 and then induced with 100 μM isopropyl β- D -1-thiogalactopyranoside and grown for 18 h at 28 °C. Cells were pelleted and resuspended in cold Tris 100 mM, MES 50 mM, acetic acid 50 mM buffer (pH 7) and then sonicated (5 × 10 s) with an ultrasonic processor VC50 sonicator (Jencons). The cleared supernatant was incubated with 1 mM Ado-Met and 1 mM MeSH in vials for 20 min before being analysed for DMS, MeSH and protein content, as above. Transcriptional assays of mddA in P. deceptionensis M1 T The sequence upstream of the P. deceptionensis M1 T mddA gene containing the predicted promoter region was cloned into the lacZ reporter plasmid pBIO1878 (ref. 46 ; Supplementary Tables 8 and 9 ). The resulting construct pBIO2232 was transformed into P. deceptionensis M1 T and transformants were grown overnight under varying conditions. Transformants were grown in the presence and absence of the potential inducer molecules 1 mM DMSP, 1 mM Met, 1 mM DMSO, 0.5 mM DMS, 0.5 mM MeSH, but also with 1 mM H 2 O 2 or 300 μM paraquat. Transformants were also incubated at 4, 15 and 28 °C; in rich versus minimal media, sulphur-limited (M9 lacking MgSO 4 ); under constant light (~50 μE m −2 s −1 ) versus dark incubation; and under aerobic versus microaerobic conditions. Finally, the cultures were assayed for β-galactosidase activities following the protocol described by Wexler et al. [47] P. deceptionensis M1 T wild type and J566 growth curves Growth curves of P. deceptionensis M1 T wild type and J566 strains were plotted for differing conditions including temperature (0 and 28 °C), salinity (NaCl 1–6%) and the absence and presence of 2 mM Met or 0.5 mM MeSH. Growth was estimated by measuring the OD 600 of the cultures at different time points using a spectrophotometer UV-1800 (Shimadzu). Oxidative stress tests For disk inhibition assays, P. deceptionensis M1 T wild type and J566 strains were grown in Mueller Hinton Broth (Oxoid) at 15 °C for 24 h and cultures adjusted to an OD 600 of 0.3. A swab was soaked in the cultures and spread onto Mueller Hinton Agar (Oxoid) plates. Sterile 6-mm filter discs (Whatman) containing 10 μl of 100 mM H 2 O 2 or 25 mM paraquat (Sigma Aldrich) were placed on the top of the plates. After an incubation period of 48 h at 15 °C, zones of growth inhibition were recorded. Minimal inhibitory concentration assays with P. deceptionensis M1 T wild type and J566 strains were performed by the broth microdilution method described by Wiegand et al. [48] using H 2 O 2 ranging from 0.4 to 100 mM or Paraquat (Sigma Aldrich) ranging from 0.1 to 25 mM. OD 600 of the wells was measured with a Synergy HT microplate reader (BioTek) after an incubation of 48 h at 15 °C. Bioinformatics analysis The protein sequence of P. deceptionensis M1 T MddA was analysed for membrane-spanning domains using the bioinformatics search engines detailed in Supplementary Table 1 . The MddA phylogenetic tree was constructed with the MEGA6 Package [49] using sequences with at least 40% amino acid identity to the MddA protein of P. deceptionensis M1 T provided by BLAST [50] . The neighbour-joining method and the Jones–Taylor–Thornton model of amino acid substitution were used, with 1,000 bootstrap replications. MddA protein sequences from P. deceptionensis M1 T (AJE75769), Pseudomonas sp. GM41 (WP_008148420.1), Cyanothece sp. ATCC 51142 (YP_001803274.1), B. diazoefficiens USDA 110 Blr1218 (NP_767858.1) and Blr5741 (NP_772381.1), Mycobacterium tuberculosis H37Rv (NP_217755.1), Maricaulis maris MCS10 (YP_757811.1), Sulfurovum sp. NBC37-1 (YP_001358232.1) and Ste14p from Saccharomyces cerevisiae (AAA16840.1) were aligned with ClustalW using the MEGA6 Package [49] and analysed for conserved domains using GeneDoc [51] v2.5.010. Ratified protein sequences of MddA (from distinct bacterial clades Figs 2 and 3 ) were used as query sequences to perform BLASTP [50] searches against peptide databases created from metagenome sequences downloaded from CAMERA and MG-RAST (information on the metagenomes is provided in Supplementary Table 4 ). The numbers of unique hits to MddA were normalized to the number of unique RecA sequences in the metagenomes to estimate the abundance of mddA in each metagenome. The number of unique RecA sequences in each metagenome was obtained using 120 RecA sequences as probes [52] ( Supplementary Table 6 ). A similar strategy was used for the DddD, L, P, Q and W sequences using ratified protein sequences as queries ( Supplementary Table 6 ). The publically available gene expression data sets for B. diazoefficiens USDA 110 and Mycobacterium tuberculosis H37Rv were analysed for conditions that resulted in significant changes in expression for the mddA gene. The B. diazoefficiens data sets were analysed using GEOR2 ( http://www.ncbi.nlm.nih.gov/geo/geo2r ). The Mycobacterium tuberculosis H37Rv data sets were analysed using the TB expression database ( http://www.tbdb.org/tbdbPages/expressionData.shtml ). Significant changes were judged as those where mddA was shown to be up- or downregulated greater than twofold in ≥2/3 of the replicates, and that were consistent at multiple time points. Accession codes: Sequence data for the cosmid pBIO2219 (accession code KM030271), the P. deceptionensis M1 T megL gene (accession code KM030270) and the P. deceptionensis M1 T MddA protein (accession code AJE75769 ) have been deposited in the NCBI GenBank database. How to cite this article: Carrión, O. et al. A novel pathway producing dimethylsulphide in bacteria is widespread in soil environments. Nat. Commun. 6:6579 doi: 10.1038/ncomms7579 (2015).